WT1 controls antagonistic FGF and BMP-pSMAD pathways in early renal progenitors Kidney organogenesis requires the tight control of proliferation, differentiation and apoptosis of renal progenitor cells. How the balance between these cellular decisions is achieved remains elusive. The Wilms’ tumour suppressor Wt1 is required for progenitor survival, but the molecular cause for renal agenesis in mutants is poorly understood. Here we demonstrate that lack of Wt1 abolishes fibroblast growth factor (FGF) and induces BMP/pSMAD signalling within the metanephric mesenchyme. Addition of recombinant FGFs or inhibition of pSMAD signalling rescues progenitor cell apoptosis induced by the loss of Wt1 . We further show that recombinant BMP4, but not BMP7, induces an apoptotic response within the early kidney that can be suppressed by simultaneous addition of FGFs. These data reveal a hitherto unknown sensitivity of early renal progenitors to pSMAD signalling, establishes FGF and pSMAD signalling as antagonistic forces in early kidney development and places WT1 as a key regulator of pro-survival FGF signalling pathway genes. In the mouse embryo, the metanephric mesenchyme (MM) forms at around embryonic day 10 as a distinct population of cells at the caudal end of the nephrogenic cord [1] . Once specified, the MM initiates a specific gene expression program, which includes the transcription factors Pax2 , Sall1 , Eya1 and Six1 , and results in the activation of the glial-derived neurotrophic factor Gdnf (ref. 1 ). Glial cell-derived neurotrophic factor (GDNF) released from the MM serves as an inductive signal that initiates ureteric budding from the nephric duct (ND). The ureteric bud (UB) subsequently invades the MM to undergo a series of dichotomous branching events giving rise to the ureteric tree. At the molecular level, GDNF binds to its tyrosine kinase receptor RET at the surface of nephric duct cells to activate an intracellular signalling cascade that includes the transcription factors Etv4 and Etv5 as the key effector genes [2] . The importance of the GDNF/RET pathway in ureter induction and growth has been demonstrated in numerous studies and the majority of knockout mouse mutants for Gdnf , its receptor Ret , and its co-receptor Gfr α 1 display renal agenesis [1] . Continuous proliferation of MM cells throughout development ensures the persistence of progenitors at the renal cortex (cap mesenchyme (CM)), whereas inductive signals initiating from the branching ureteric tree promote the adjacent MM cells to undergo differentiation into epithelial nephrons [1] . The maintenance of undifferentiated renal progenitor cells is under control of the transcription factor SIX2 (refs 3 , 4 ). Additional factors required for MM survival have long been unknown, but recently a series of experiments has implicated the fibroblast growth factor (FGF) pathway in self-renewal [5] , [6] . Indeed, mutations in FGF20 have been identified in patients with renal agenesis and simultaneous deletion of Fgf20 and Fgf9 results in apoptosis of the MM in the mouse [7] . However, the molecular mechanism triggering correct expression of FGFs during kidney organogenesis remains unknown. Wt1 encodes a zinc-finger transcription factor that has been identified as a gene mutated in Wilms’ tumour, a paediatric kidney tumour that is believed to arise from renal progenitor cells [8] . Wt1 expression is found within the early MM, persists within renal progenitors throughout development and is also found within the proximal part of forming nephrons [9] . Wt1 deletion in mice results in bilateral renal agenesis characterized by a failure of the ureteric bud to completely form and concurrent apoptosis of the MM [10] . In vitro tissue recombination experiments demonstrate that isolated Wt1 knockout MM fails to survive even when recombined with a wild-type ureter indicating that WT1 is required intrinsically within the MM cells [11] . Genetic experiments in mice further revealed additional requirements for WT1 in mesenchymal to epithelial transition (MET) [12] , [13] and podocyte maturation [14] . Although direct downstream targets of WT1 in kidney development have been identified in the past [15] , a clear link between these target genes and the renal agenesis phenotype has not been established. Here we use a combination of chromatin immunoprecipitation-sequencing (ChIP-Seq), microarray and functional studies to demonstrate that WT1 is required to suppress BMP/pSMAD and induce FGF signalling in the early kidney anlagen. ChIP-Seq analysis identifies genome-wide WT1-binding sites We performed in vivo ChIP-Seq analysis on E18.5 kidneys using a modified ChIP-Seq protocol to obtain an unbiased view of WT1-bound regions throughout the genome. Two independent experiments were carried out that provided highly similar results ( Supplementary Fig. 1 ) and were therefore used as replicates for bioinformatic analysis. Mapping of sequenced tags using the Genomatix Genome Analyzer identified 36,512 enriched clusters that showed an enrichment of peaks within promoter regions of 4.9-fold for all ( Fig. 1 ; Supplementary Fig. 1 ; Supplementary Data 1 ). Irreproducibility Discovery Rate (IDR) analysis [16] with an IDR cutoff of ≤0.1 and ≤0.01 yielded 5,547 and 2,940 peaks, respectively, ( Supplementary Data 2 ). Using peaks with an IDR below 0.01, MEME-ChIP analysis [17] , [18] identified a highly enriched binding motif (E-value=1.1e−120, expected number of motifs with the given minimum log likelihood ratio) with significant similarity to the WT1 motif previously identified from ChIP-on-Chip experiments [15] (top match, E-value=0.002; Bonferroni corrected P -value; Fig. 1a ) closely followed by the motifs for the zinc-finger proteins EGR2 (E-value=0.003; Bonferroni corrected P -value) and EGR1 (E-value=0.006; Bonferroni corrected P -value). 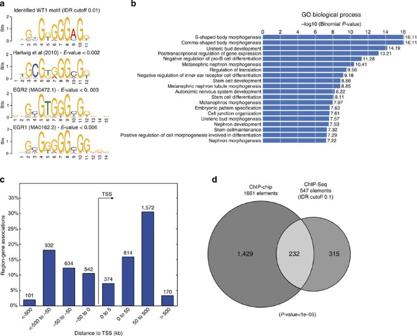Figure 1: ChIP-Seq analysis definesin vivobinding sites for WT1 in kidney development. (a) Logo representations of the identified WT1-binding motif showing significant similarity to the WT1 motif discovered by ChIP-on-Chip15and other members of the EGR family of transcription factors. (b) Functional annotation of peaks with IDR<0.01 (Genomic Regions Enrichment of Annotations Tool (GREAT) analysis) revealed a strong enrichment of targets involved in kidney development. (c) Mapping of peaks with IDR<0.01 suggests that WT1 is predominately working through distal regulatory elements. (d) Comparison of the 547 genes with ChIP-Seq peaks within 5.5 kb upstream and 2.5 kb downstream of the transcription start site with the list of 1,661 targets identified by ChIP-on-Chip analysis15revealed a significant overlap of 232 genes. Figure 1: ChIP-Seq analysis defines in vivo binding sites for WT1 in kidney development. ( a ) Logo representations of the identified WT1-binding motif showing significant similarity to the WT1 motif discovered by ChIP-on-Chip [15] and other members of the EGR family of transcription factors. ( b ) Functional annotation of peaks with IDR<0.01 (Genomic Regions Enrichment of Annotations Tool (GREAT) analysis) revealed a strong enrichment of targets involved in kidney development. ( c ) Mapping of peaks with IDR<0.01 suggests that WT1 is predominately working through distal regulatory elements. ( d ) Comparison of the 547 genes with ChIP-Seq peaks within 5.5 kb upstream and 2.5 kb downstream of the transcription start site with the list of 1,661 targets identified by ChIP-on-Chip analysis [15] revealed a significant overlap of 232 genes. Full size image Genomic Regions Enrichment of Annotations Tool (GREAT) analysis [18] was used to perform functional annotation on peaks in relation to transcription start sites (TSSs). Peak-associated genes (IDR cutoff 0.01) showed a clear enrichment in kidney development with S-shaped body morphogenesis, comma-shaped body morphogenesis and ureteric bud development being the top three hits for gene ontology (GO) biological processes ( Fig. 1b ). Genes associated with WT1-ChIP peaks exhibit expression patterns (according to GUDMAP ( www.gudmap.org [19] ) and Eurexpress ( www.eurexpress.org ) databases) overlapping with that of Wt1 with a proportion of targets showing restriction to the early MM (for example, Hoxb1 ; P =9.99e−80; Bonferroni corrected P -value), the renal vesicle (for example, Heyl; P =3.51e−32; Bonferroni corrected P -value) or podocytes (for example, Pard6B ; P =7.01e−95; Bonferroni corrected P -value). Comparison of peak-associated genes with molecular signature databases (MSigDB) revealed as top hit a gene set found to be induced upon WT1 expression [20] ( Supplementary Fig. 1C ). We next mapped WT1-binding sites with respect to TSS of WT1-associated genes. Interestingly, only about 20% of WT1-binding sites were within 5 kb of any TSS, while >50% are located 50–500 kb from the closest TSS ( Fig. 1c ). These results suggest that WT1 may predominantly work through distal regulatory elements rather than by direct binding to promoter regions. We next compared our data set with the list of genes previously identified as WT1 targets using ChIP-on-Chip analysis [15] . Oligos on the tiling arrays were used for this publication cluster −5.5 kb and +2.5 kb around the TSS of genes, and we therefore selected only genes associated with peaks falling within these regions. List comparison revealed an overlap of 232 genes (42%) between ChIP-Seq and ChIP-on-Chip data (random sampling out of the ChIP-on-Chip pool of 17,296 genes with subsequent assessment of the set intersection, P -value <1e−05) ( Fig. 1d ; Supplementary Data 3 ). WT1 controls a subset of renal progenitor-specific genes Identification of WT1-bound regions provides a framework of genes that are potentially regulated by WT1, but does not necessarily imply clear-cut functional relationships. To identify genes whose expression depends on WT1 at the onset of metanephric kidney organogenesis, we carried out microarray-based gene expression profiling at E10.25 ( Fig. 2a ), a time point before the onset of apoptosis in Wt1 mutants ( Supplementary Fig. 2A ). Setting a P -value cutoff at <0.05 and a raw data value cutoff of 1,000 identified 34 and 88 genes with >twofold change induced or reduced expression, respectively ( Supplementary Data 4 ). Differential gene expression of selected WT1 target genes was confirmed by quantitative PCR (qPCR) analysis and whole-mount in situ hybridization (WISH) ( Fig. 2b,c ). One exception was Six2 for which qPCR analysis revealed no significant change, and antibody staining on E10.25 embryos confirmed persistence of expression in Wt1 mutant MM ( Supplementary Fig. 9 ). Probing public databases of mouse in situ hybridization data sets (GUDMAP, Eurexpress) and our own in situ hybridization analysis ( Fig. 2d ; Supplementary Fig. 2C ) confirmed that many downregulated genes were indeed enriched within the renal progenitor compartment. 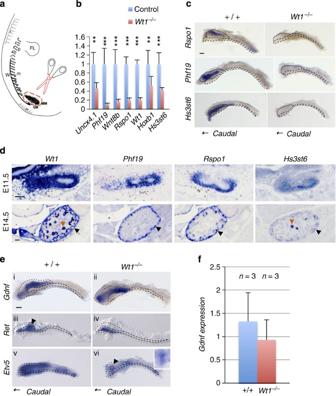Figure 2: Gene expression profiling reveals a set of WT1-dependent genes expressed in the cap mesenchyme. (a) Schematic representation of the microsurgical isolation of metanephric kidney anlagen for microarray analysis. (b) qPCR confirmation of genes downregulated inWt1mutant kidney anlagen. Sample sizen=4. Error bars represent s.e.m.P-values of ≤0.01 and 0.001 (Student’st-tests) are indicated with ** and ***, respectively. (c) WMISH analysis (E10.25) demonstrating loss ofRspo1,Phf19andHs3st6gene expression in the mesenchymal compartment ofWt1mutant kidney rudiments. (d)In situhybridization on sagittal sections of wild-type embryos. At E11.5,Wt1,Phf19,Rspo1andHs3st6are strongly expressed in the mesenchymal tissue surrounding the epithelial T-stage ureter. At E14.5, three classes of gene expression patterns were observed: (1) expression restricted to renal progenitors (black arrowheads), as exemplified byPhf19. Note that gene expression is confined to the renal cortex. (2) Expression in both renal progenitors and early nephrogenic stages (for example,Rspo1). Expression is absent from differentiated podocytes. (3) Expression in renal progenitors and differentiated glomerular podocytes (orange arrowheads) as illustrated byWt1andHs3st6. (e) Whole-mountin situhybridization on E10.25 urogenital ridges demonstrates persistence ofGdnfandRetexpression within mutant MM (dotted lines) and mesonephric ducts (dashed lines). The GDNF/RET effectorEtv5is considerably reduced in mutant MM. Note the induction ofEtv5in the epithelial bud in those mutants where initial induction occurs (inset in vi). (c–e) Scale bar, 100 μm. (f) Quantification ofGdnfRNA levels by qPCR confirms no significant change of expression levels inWt1mutant animals. The number of biological replicates (n) is given above each bar. Figure 2: Gene expression profiling reveals a set of WT1-dependent genes expressed in the cap mesenchyme. ( a ) Schematic representation of the microsurgical isolation of metanephric kidney anlagen for microarray analysis. ( b ) qPCR confirmation of genes downregulated in Wt1 mutant kidney anlagen. Sample size n =4. Error bars represent s.e.m. P -values of ≤0.01 and 0.001 (Student’s t -tests) are indicated with ** and ***, respectively. ( c ) WMISH analysis (E10.25) demonstrating loss of Rspo1 , Phf19 and Hs3st6 gene expression in the mesenchymal compartment of Wt1 mutant kidney rudiments. ( d ) In situ hybridization on sagittal sections of wild-type embryos. At E11.5, Wt1 , Phf19 , Rspo1 and Hs3st6 are strongly expressed in the mesenchymal tissue surrounding the epithelial T-stage ureter. At E14.5, three classes of gene expression patterns were observed: (1) expression restricted to renal progenitors (black arrowheads), as exemplified by Phf19 . Note that gene expression is confined to the renal cortex. (2) Expression in both renal progenitors and early nephrogenic stages (for example, Rspo1 ). Expression is absent from differentiated podocytes. (3) Expression in renal progenitors and differentiated glomerular podocytes (orange arrowheads) as illustrated by Wt1 and Hs3st6 . ( e ) Whole-mount in situ hybridization on E10.25 urogenital ridges demonstrates persistence of Gdnf and Ret expression within mutant MM (dotted lines) and mesonephric ducts (dashed lines). The GDNF/RET effector Etv5 is considerably reduced in mutant MM. Note the induction of Etv5 in the epithelial bud in those mutants where initial induction occurs (inset in vi). ( c – e ) Scale bar, 100 μm. ( f ) Quantification of Gdnf RNA levels by qPCR confirms no significant change of expression levels in Wt1 mutant animals. The number of biological replicates ( n ) is given above each bar. Full size image Comparison of our data with previous microarray studies performed on gonadal ridges [21] or adult kidneys [22] from Wt1 mutant animals revealed little overlap ( Supplementary Fig. 2B ), indicating that gene sets regulated by WT1 largely depend on tissue context. Examination of the genomic loci of the top 15 downregulated genes (by fold change) identified clear WT1-bound regions (peaks) in the proximity of the TSS of 11 of them ( Supplementary Fig. 3 ). A graphical view and a complete list of peaks mapping in proximity to genes deregulated in Wt1 mutants are provided in Supplementary Fig. 4 and Supplementary Data 5 , respectively. Taken together these data suggest that a large proportion of the genes identified in the microarray screen are directly bound by WT1. Annotation clustering using GOrilla [23] identified 35 processes satisfying a P -value <e−04 (minimum hypergeometric score) with metanephros development (3rd position; P -value 1.12e−07) scoring an eightfold enrichment ( Supplementary Data 6 ). Since ureteric bud development also scored highly (sevenfold enrichment) and the receptor tyrosine kinase downstream targets Etv5 (3.4-fold; P =7.4e−06; Welch parametric t -test) [2] , Dusp6 (twofold; P =9.7e−07; Welch parametric t -test) and Cxcr4 (2.1-fold; P =6.6e−04; Welch parametric t -test) were downregulated ( Supplementary Data 4 ), we tested a potential disruption of GDNF signalling in Wt1 mutant animals. WISH and qPCR analysis, however, revealed persistence of GDNF/RET signalling and activation of its target Etv5 ( Fig. 2e,f ) in the epithelial compartment, a finding that is consistent with earlier studies [11] . Interestingly, mesenchymal Etv5 expression was markedly reduced indicating severe defects in receptor tyrosine kinase signalling in this compartment ( Fig. 2e ). WT1 induces FGF expression within the developing kidney The FGF pathway was the top enriched cluster (28 × enrichment, FDR 2.7e−04; (ref. 23 )), when choosing ‘Function’ as ontology in GOrilla analysis ( Supplementary Fig. 5 ). This suggested that regulation of FGF signalling might represent an essential function of WT1 during early kidney organogenesis. Indeed, our gene expression profiling studies revealed reduced expression of several Fgf genes in Wt1 knockout tissue including Fgf8 (2.2-fold), Fgf10 (2.8-fold), Fgf16 (2.1-fold), Fgf18 (2.3-fold) and Fgf20 (3.4–fold). Reduced Fgf gene expression was confirmed independently by qPCR assays (downregulation of Fgf8= 2.3-fold; P =0.01; Fgf10 =2.1-fold; P =5.1e−05; Fgf16 =1.7-fold; P =0.07; Fgf18 =1.7; P =0.009; Fgf20 =3.5-fold; P =2.4e−05; sample size n =4; Student’s t -test). Analysis of genomic regions identified specific WT1-bound ChIP-Seq peaks in the promoters of Fgf16 (IDR=0.0058) and Fgf20 (IDR=1.245e−5) and upstream of Fgf8 (IDR=0.0027) ( Fig. 3a ; Supplementary Data 1 ). Fgf20 is known to be expressed within the MM, where it fulfills an important function in progenitor proliferation [7] . Fgf16 , while detectable by qPCR analysis, did not reveal a clear signal in ISH experiments, suggesting that expression of this gene in the early MM must be low. 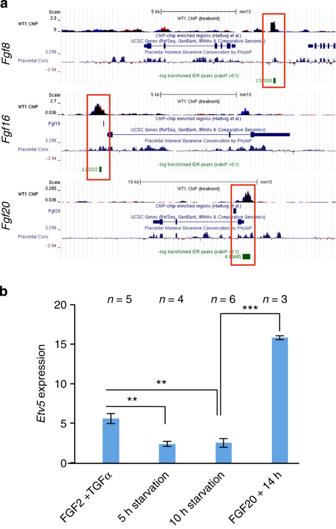Figure 3: FGF signalling in MM depends on WT1. (a) ChIP-Seq analysis on E18.5 kidneys identifies direct binding of WT1 close to the loci ofFgf8(IDR=0.0027),Fgf16(IDR=0.0058) andFgf20(IDR=1.2454e−5). Upper tracks were generated by overlaying the two independent WT1-ChIP-Seq data sets (red and blue, regions with overlap are depicted in black). ChIP-on-Chip-defined WT1-binding sites, where present, are shown as vertical bars in the second track. Evolutionary conservation is depicted below the genes. WT1-ChIP-enriched regions are shown as green vertical bars with their respective IDR and highlighted with a red rectangle. (b)Etv5expression is activated by FGF signalling. Starving of isolated MM (E11.5, dissociated from the ureter) leads to loss ofEtv5expression. Addition of FGF20 results in eightfold increase of RNA levels. ***P<0.001, **P<0.01 using the Student’st-test. Error bars represent s.e.m. The number of biological replicates (n) is given above each bar. Figure 3: FGF signalling in MM depends on WT1. ( a ) ChIP-Seq analysis on E18.5 kidneys identifies direct binding of WT1 close to the loci of Fgf8 (IDR=0.0027), Fgf16 (IDR=0.0058) and Fgf20 (IDR=1.2454e−5). Upper tracks were generated by overlaying the two independent WT1-ChIP-Seq data sets (red and blue, regions with overlap are depicted in black). ChIP-on-Chip-defined WT1-binding sites, where present, are shown as vertical bars in the second track. Evolutionary conservation is depicted below the genes. WT1-ChIP-enriched regions are shown as green vertical bars with their respective IDR and highlighted with a red rectangle. ( b ) Etv5 expression is activated by FGF signalling. Starving of isolated MM (E11.5, dissociated from the ureter) leads to loss of Etv5 expression. Addition of FGF20 results in eightfold increase of RNA levels. *** P <0.001, ** P <0.01 using the Student’s t -test. Error bars represent s.e.m. The number of biological replicates ( n ) is given above each bar. Full size image As described above, we observed loss of Etv5 expression in the mesenchymal compartment of Wt1 knockout embryos. Since this gene has been reported to be a downstream target of FGF signalling in other organ systems [24] , we asked whether Etv5 might be also in the kidney under direct control of this pathway. To address this question, we isolated MM from E11.5 embryos and expanded primary cultures in medium containing FGF2 and transforming growth factor alpha, as previously defined [25] . Subsequent culturing in serum free medium (for 5 or 10 h) resulted in a threefold reduction of Etv5 expression ( Fig. 3b ). Strikingly, addition of FGF20 after starvation induced Etv5 expression eightfold indicating a clear dependence of this gene on FGF signalling. Recombinant FGF rescues apoptosis caused by loss of Wt1 FGF signalling is implicated in MM progenitor survival/proliferation [6] and we asked whether exogenous FGFs would be sufficient to rescue mesenchymal apoptosis caused by loss of Wt1 . We first employed a gene knockdown approach [15] by culturing E11.5 kidney cultures in the presence of Vivo-Morpholinos . Test experiments confirmed the suitability of such an approach and oligos targeting Wnt4 resulted in a significant reduction in number of renal vesicles (marked by JAG1) within the developing organoid ( Supplementary Fig. 6A,B ), a phenotype that is consistent with the established function of Wnt4 in MET and early nephrogenesis [26] . When treating kidney explants with Vivo-Morpholino targeting Wt1 , cultures stopped branching and mesenchymal cells underwent massive apoptosis ( Fig. 4a ; Supplementary Fig. 6C ), thus phenocopying the defects in Wt1 knockout mice [10] . Antibody staining of Wt1 Vivo-Morpholino -treated tissue samples confirmed a marked reduction of WT1, but persistence of a small number of PAX2- and SIX2-positive cells ( Supplementary Fig. 6C ). Addition of an antimer (reverse complement oligonucleotide to the Wt1 Vivo-Morpholino ) effectively blocked morpholino action and kidney cultures developed normally, thus ruling out unspecific toxicity effects of the added Vivo - Morpholino ( Supplementary Fig. 6C ). 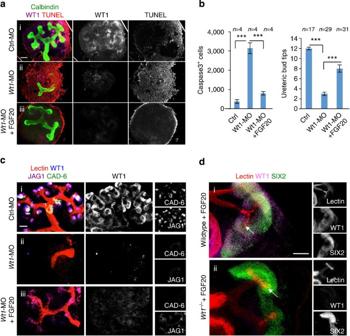Figure 4: Recombinant FGF20 rescues renal defects induced by loss of WT1. (a)Wt1knockdown in E11.5 kidney cultures usingVivo-Morpholinosphenocopies the renal deficiencies observed inWt1mutant mice with a marked increase of apoptosis and loss of ureter branching after 48 h in culture. Addition of FGF20 (5 ng ml−1) to the culture medium rescues both apoptosis and branching defects. (b) Quantification of caspase 3-positive (apoptotic) cells and ureteric tips in independent rescue experiments. ***P<0.001; Student’st-test. Error bars represent s.e.m. The number of biological replicates (n) is given above each bar. (c) Long term cultures (72 h) reveal that addition of recombinant FGF20 complements growth defects induced byWt1knockdown, but does not rescue MET defects, as evidenced by an almost complete absence of JAG1-(violet) and cadherin-6 (green)-positive renal vesicles (iii). (d) Addition of recombinant FGF20 (50 ng ml−1) to urogenital ridge cultures (isolated at E10.25 and cultured for 72 h) rescues renal defects inWt1knockout embryos. Note the presence of a T-shaped ureter (arrow) and persistence of SIX2-positive cap mesenchyme (asterisk) despite the absence of WT1. Scale bar, 100 μm. Figure 4: Recombinant FGF20 rescues renal defects induced by loss of WT1. ( a ) Wt1 knockdown in E11.5 kidney cultures using Vivo-Morpholinos phenocopies the renal deficiencies observed in Wt1 mutant mice with a marked increase of apoptosis and loss of ureter branching after 48 h in culture. Addition of FGF20 (5 ng ml −1 ) to the culture medium rescues both apoptosis and branching defects. ( b ) Quantification of caspase 3-positive (apoptotic) cells and ureteric tips in independent rescue experiments. *** P <0.001; Student’s t -test. Error bars represent s.e.m. The number of biological replicates ( n ) is given above each bar. ( c ) Long term cultures (72 h) reveal that addition of recombinant FGF20 complements growth defects induced by Wt1 knockdown, but does not rescue MET defects, as evidenced by an almost complete absence of JAG1-(violet) and cadherin-6 (green)-positive renal vesicles (iii). ( d ) Addition of recombinant FGF20 (50 ng ml −1 ) to urogenital ridge cultures (isolated at E10.25 and cultured for 72 h) rescues renal defects in Wt1 knockout embryos. Note the presence of a T-shaped ureter (arrow) and persistence of SIX2-positive cap mesenchyme (asterisk) despite the absence of WT1. Scale bar, 100 μm. Full size image Next, we added recombinant FGF proteins to kidney organ cultures to test whether they are sufficient to rescue the Wt1 morphant phenotypes. Addition of 5 ng ml −1 FGF20 or 50 ng ml −1 FGF10 medium had no discernible effect on renal growth in the presence or absence of control Vivo-Morpholino ( Supplementary Fig. 7A ). In contrast, apoptosis and branching defects caused by Wt1 Vivo-Morpholino were largely rescued in explants treated with FGF20 ( n =31/47) or FGF10 ( n =3/3) ( Fig. 4a,b ; Supplementary Fig. 7B,C ). Importantly, mesenchymal cells maintained their condensed appearance and the significant reduction of terminal deoxynucleotidyl transferase dUTP nick end labelling (TUNEL)/caspase 3-positive cells indicated that they had escaped apoptosis ( Fig. 4a,b ; Supplementary Fig. 7B ). Similar results were obtained with Wt1 CreERT2 /Wt1 flox/flox organ cultures after tamoxifen-induced deletion of Wt1 and following FGF treatment ( Supplementary Fig. 7D ). Thus, irrespective of the gene-silencing method used, addition of exogenous FGFs rescues WT1-deficient kidney explants from apoptosis. WT1 acts at multiple stages during kidney development and we wanted to examine to what extent exogenous FGF20 could support renal growth and differentiation in the absence of WT1. Kidneys treated with Wt1 Vivo - Morpholino failed to recover in FGF-free media even after 72 h and cultures almost completely lacked mesenchymal tissues ( Fig. 4c ). In contrast, addition of FGF20 led to sustained growth of organ cultures with rescued samples showing some degree of phenotypic variation dependent on the efficacy of the WT1 knockdown. In samples in which low levels of WT1 persisted (incomplete knockdown), some MET occurred, as evidenced by the expression of JAG1 and cadherin-6, two markers of early renal vesicles ( Supplementary Fig. 7C ). On the other hand, cultures with a complete knockdown of WT1, lacked renal vesicles ( Fig. 4c ), an observation that is consistent with a role for WT1 in MET [12] , [13] . The potential direct regulation by WT1 of Fgf8 ( Fig. 3a ) and Wnt4 (ref. 12 ), two genes required for MET, provides a molecular explanation for this phenotype. Finally, we tested whether addition of FGF20 would also be sufficient to rescue E10.25 cultures of Wt1 knockout ( Wt1 −/− ) urogenital ridges. Wild-type cultures showed a T-branched ureter surrounded by SIX2- and WT1-positive cells after 48 h of culture ( Supplementary Fig. 7E ). In contrast, SIX2 + cells were absent from Wt1 −/− urogenital ridges and the ureteric bud failed to grow out ( Supplementary Fig. 7E ). Addition of 50 ng ml −1 of FGF20 to the culture medium had little effect on growth and differentiation of wild-type cultures ( Fig. 4d i), although we noticed the formation of anterior ectopic buds in a proportion of cultures. Strikingly, FGF20 rescued early kidney development of Wt1 −/− explants and SIX2 + MM cells persisted despite the absence of WT1 ( Fig. 4d ii). Inhibition of pSMAD signalling suppresses apoptosis Our microarray analysis not only revealed decreased FGF signalling, but also showed an increase of Msx1 (twofold; P =0.006; Welch parametric t -test) and Tbx5 (2.5-fold; P =0.002; Welch parametric t -test) expression ( Supplementary Data 4 ), two known downstream targets of BMP4 signalling [27] , [28] . Binding of WT1 to Bmp4 and Bmp7 has been reported previously( [15] and this study), but expression of these genes is not changed in E10.25 Wt1 mutants ( Supplementary Data 4 ). In addition, kidneys develop normally until E13.5 in Bmp7 mutants [29] and it is therefore unlikely that this gene directly contributes to the early renal agenesis phenotype in Wt1 knockout mice. However, expression of Bmper (Cv2) , a direct target of WT1 ( Fig. 5b ; Supplementary Data 1 ; IDR=0.008) that can act as a positive and negative modifier of BMP signalling [30] , was reduced 2.2-fold ( P =3.4e−6; Student’s t -test) in Wt1 -deficient kidney anlagen ( Supplementary Data 4 ). In addition, Wt1 knockdown experiments confirmed loss of Bmper expression as early as 24 h after Vivo-Morpholino treatment ( Supplementary Fig. 8 ). 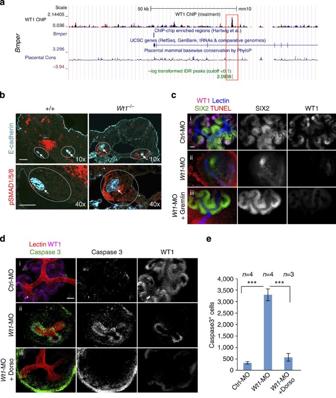Figure 5: Inhibition of BMP/pSMAD signalling reverts renal defects induced byWt1knockdown. (a) ChIP-Seq analysis identifies direct binding of WT1 within intron 3 of the BMP inhibitorBmper(IDR=0.008). Upper tracks were generated by overlaying the two independent WT1-ChIP-Seq data sets (red and blue, regions with overlap are depicted in black). The ChIP-on-Chip-identified WT1-binding site is shown as a vertical bar in the second track. Evolutionary conservation is depicted below the genes. Wt1-ChIP-enriched regions are shown as green vertical bars with their respective IDR and highlighted with a red rectangle. (b) Immunofluorescent analysis at E10.5 reveals a massive increase of phospho-SMAD staining (pSMAD1/5/8 in red) inWt1mutant MM, when compared with wild-type embryos. The epithelial marker E-cadherin (blue) outlines the nephric ducts (arrows). The red signal marked by an asterisk (control samples) represents blood cells trapped within the dorsal aorta. (c) Addition of the BMP inhibitor Gremlin reverts apoptosis induced by WT1Vivo-Morpholinoknockdown in organ cultures. (d) Addition of the pSMAD pathway-specific inhibitor dorsomorphin (Dorso) rescued apoptosis induced byWt1knockdown. (e) Quantification of caspase 3 (apoptotic) pictured in panele. ***P<0.001 using the Student’st-test. Error bars represent s.e.m. Scale bar, 100 μm. The number of biological replicates (n) is given above each bar. Figure 5: Inhibition of BMP/pSMAD signalling reverts renal defects induced by Wt1 knockdown. ( a ) ChIP-Seq analysis identifies direct binding of WT1 within intron 3 of the BMP inhibitor Bmper (IDR=0.008). Upper tracks were generated by overlaying the two independent WT1-ChIP-Seq data sets (red and blue, regions with overlap are depicted in black). The ChIP-on-Chip-identified WT1-binding site is shown as a vertical bar in the second track. Evolutionary conservation is depicted below the genes. Wt1-ChIP-enriched regions are shown as green vertical bars with their respective IDR and highlighted with a red rectangle. ( b ) Immunofluorescent analysis at E10.5 reveals a massive increase of phospho-SMAD staining (pSMAD1/5/8 in red) in Wt1 mutant MM, when compared with wild-type embryos. The epithelial marker E-cadherin (blue) outlines the nephric ducts (arrows). The red signal marked by an asterisk (control samples) represents blood cells trapped within the dorsal aorta. ( c ) Addition of the BMP inhibitor Gremlin reverts apoptosis induced by WT1 Vivo - Morpholino knockdown in organ cultures. ( d ) Addition of the pSMAD pathway-specific inhibitor dorsomorphin ( Dorso ) rescued apoptosis induced by Wt1 knockdown. ( e ) Quantification of caspase 3 (apoptotic) pictured in panel e . *** P <0.001 using the Student’s t -test. Error bars represent s.e.m. Scale bar, 100 μm. The number of biological replicates ( n ) is given above each bar. Full size image To test whether BMP signalling is indeed activated in mutant mesenchyme, we performed immunostaining with antibodies recognizing the phosphorylated version of SMAD1/5/8 (pSMAD1/5/8), the downstream effectors of canonical BMP signalling [31] . While wild-type and Wt1 heterozygous mutant MM were largely devoid of pSMAD1/5/8 staining at E10.5, sections of mutant embryos showed a marked increase of nuclear staining in mesenchymal cells surrounding the mesonephric duct including the SIX2-positive population ( Fig. 5b ; Supplementary Fig. 9 ). We next tested whether inhibition of BMP signalling may complement loss of Wt1 function. Addition of recombinant Gremlin, an inhibitor of BMP signalling, partially rescued the WT1 Vivo - Morpholino knockdown phenotype ( Fig. 5c ) albeit to a lower extent than FGF20. Furthermore, treatment with the pSMAD-specific inhibitor dorsomorphin [32] efficiently suppressed Wt1 Vivo - Morpholino -induced apoptosis within the CM and the kidney cultures underwent successive rounds of branching ( Fig. 5d,e ). We conclude that loss of WT1 within the early kidney anlagen directly impacts FGF gene expression and enhances canonical BMP signalling, and that inhibition of BMP/pSMAD signalling is sufficient to permit MM survival. BMP4 but not BMP7 induces apoptosis in early kidney explants BMP signalling is widely considered as a pro-survival factor in MM cells and Bmp7 knockout mice show a premature exhaustion of the renal progenitor pool [29] . Our observation that loss of Wt1 can be rescued by inhibition of the BMP pathway seems surprising and we wondered whether the cellular response might depend on the type of BMP ligand. Addition of recombinant BMP7 to E11.5 kidney organ cultures had little effect on renal development and, if at all, increased overall growth ( Fig. 6c ). In contrast, addition of BMP4 resulted in massive apoptosis of MM progenitor cells and a complete block of development ( Fig. 6a,b ) an observation already made in an earlier study [33] . This striking effect was observed even at very low concentrations of BMP4 (1 ng to 400 ng ml −1 ). Addition of recombinant Gremlin, BMPER or dorsomorphin reverted the BMP4-induced apoptosis phenotype indicating that this phenotype is BMP4 specific and involves pSMAD signalling ( Fig. 6a,b ; Supplementary Fig. 10 ). 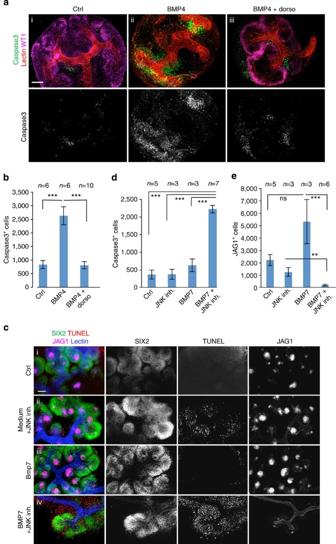Figure 6: BMP4 and BMP7 induce distinct responses in early renal explants. (a) Addition of recombinant BMP4 (40 ng ml−1) to kidney cultures caused massive apoptosis and kidneys failed to develop (compare i and ii). Simultaneous addition of the pSMAD inhibitor dorsomorphin (5 μM) reverted the phenotype (iii). (b) Quantification of caspase 3-positive cells after 48 h in culture. (c) Culturing kidneys in the presence of the JNK pathway inhibitor S600125 (10 μM) caused an increase of the number of apoptotic cells, but did not interfere with organ growth (compare i and ii). Addition of recombinant BMP7 (400 ng ml−1) had little effect on overall renal growth (iii). Simultaneous addition of recombinant BMP7 and the JNK pathway inhibitor S600125 caused massive apoptosis and cultures failed to develop (iv). (d) Quantification of caspase3-positive cells inc. (e) Quantification of JAG1-positive cells inc. (see alsoSupplementary Fig. 6). ***P<0.001, **P<0.01; Student’st-test. Error bars represent s.e.m. Scale bar, 100 μm. The number of biological replicates (n) is given above each bar. NS, not significant. Figure 6: BMP4 and BMP7 induce distinct responses in early renal explants. ( a ) Addition of recombinant BMP4 (40 ng ml −1 ) to kidney cultures caused massive apoptosis and kidneys failed to develop (compare i and ii). Simultaneous addition of the pSMAD inhibitor dorsomorphin (5 μM) reverted the phenotype (iii). ( b ) Quantification of caspase 3-positive cells after 48 h in culture. ( c ) Culturing kidneys in the presence of the JNK pathway inhibitor S600125 (10 μM) caused an increase of the number of apoptotic cells, but did not interfere with organ growth (compare i and ii). Addition of recombinant BMP7 (400 ng ml −1 ) had little effect on overall renal growth (iii). Simultaneous addition of recombinant BMP7 and the JNK pathway inhibitor S600125 caused massive apoptosis and cultures failed to develop (iv). ( d ) Quantification of caspase3-positive cells in c . ( e ) Quantification of JAG1-positive cells in c . (see also Supplementary Fig. 6 ). *** P <0.001, ** P <0.01; Student’s t -test. Error bars represent s.e.m. Scale bar, 100 μm. The number of biological replicates ( n ) is given above each bar. NS, not significant. Full size image The pro-proliferative action of BMP7 on MM has been attributed to the activation of c-Jun N-terminal kinase (JNK)- rather than pSMAD signalling [34] . To test whether JNK inhibition would affect BMP action, we added the small-molecule inhibitor SP60015 to our organ cultures. Treatment of kidneys with 10 μM SP60015 only marginally affected explant growth, although TUNEL and Caspase 3 staining revealed some mesenchymal apoptosis ( Fig. 6cii,d ). Simultaneous treatment of cultures with recombinant BMP7 and SP60015, however, induced widespread apoptosis and kidneys failed to develop under these conditions ( Fig. 6civ,d,e ). JNK inhibition did not alter the effect of BMP4, and cultures rapidly underwent apoptosis. Thus, the early MM responds differentially to BMPs: BMP7 acts pro-proliferative, whereas BMP4 induces apoptosis. Inhibition of JNK signalling by SP60015 appears to transform the effect of BMP7 from pro-proliferative to pro-apoptotic, thus eliciting now an activity comparable to BMP4. FGF20 suppresses BMP4-induced apoptosis The apparent opposing effects of FGF20 and BMP4 on early kidney development and the fact that FGF20 was able to rescue apoptosis of MM in Wt1 −/− embryos prompted us to assess the epistatic relationship of these two signalling molecules. As described above, treatment of cultures with BMP4 (25 ng ml −1 ) induced massive apoptosis in the CM of E11.5 kidney explants ( Fig. 7aii,b ). Strikingly, simultaneous treatment of cultures with BMP4 and FGF20 (20 ng ml −1 ) inhibited the apoptotic response of explants and permitted survival of WT1-positive progenitor cells ( Fig. 7aiii,b ). 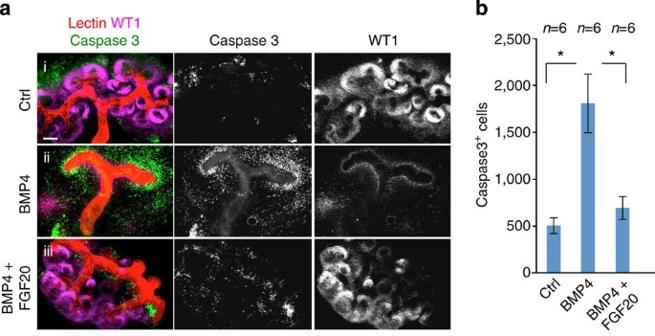Figure 7: Antagonistic action of FGF and BMP pathways in early kidney explants. (a) Addition of recombinant FGF20 rescued MM apoptosis induced by BMP4 and permitted growth and differentiation of WT1-positive progenitor cells (compare ii and iii). (b) Quantification of caspase 3-positive cells in six independent samples confirms suppression of BMP4-induced apoptosis by FGF20. *P<0.05; Student’st-test. Error bars represent s.e.m. Scale bar, 100 μm. The number of biological replicates (n) is given above each bar. Figure 7: Antagonistic action of FGF and BMP pathways in early kidney explants. ( a ) Addition of recombinant FGF20 rescued MM apoptosis induced by BMP4 and permitted growth and differentiation of WT1-positive progenitor cells (compare ii and iii). ( b ) Quantification of caspase 3-positive cells in six independent samples confirms suppression of BMP4-induced apoptosis by FGF20. * P <0.05; Student’s t -test. Error bars represent s.e.m. Scale bar, 100 μm. The number of biological replicates ( n ) is given above each bar. Full size image To test whether suppression of pSMAD activity is a normal function of FGF during kidney development, we used FGF pathway inhibitors in organ cultures. Addition of the FGF receptor inhibitor SU5402 had marked effects on explant growth, and cultures underwent apoptosis within 24–48 h after treatment ( Fig. 8a ). pSMAD staining in control explants was restricted to a small number of cells that are primed for MET [35] , whereas inhibition of FGF signalling resulted in widespread activation of pSMAD throughout the explant ( Fig. 8a ). 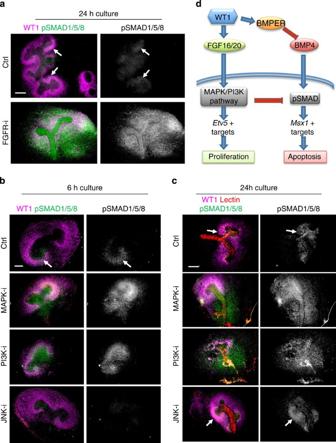Figure 8: FGF signalling is required to suppress pSMAD signalling in early kidney development. (a) Addition of the FGF receptor inhibitor SU5402 to E11.5 kidney explants inhibited growth and branching and resulted in widespread activation of pSMAD1/5/8. (b,c) The MAPK inhibitor U0126 and PI3K inhibitor LY294002 induced apoptosis as early as 6 h after addition to cultures. In contrast, addition of the JNK pathway inhibitor SP600125 had little effect on tissue growth. (d) Working model of signalling pathways regulated by WT1 in early MM. WT1 induces FGF signalling by directly regulatingFgf16andFgf20gene expression. Binding of FGF to its receptors activates intracellular signalling pathways that induce proliferation and directly suppress pSMAD signalling. In the absence of WT1, loss of FGF signalling and the induction of the BMP/pSMAD signalling pathway leads to widespread apoptosis within the metanephric blastema. Scale bar, 100 μm. Figure 8: FGF signalling is required to suppress pSMAD signalling in early kidney development. ( a ) Addition of the FGF receptor inhibitor SU5402 to E11.5 kidney explants inhibited growth and branching and resulted in widespread activation of pSMAD1/5/8. ( b , c ) The MAPK inhibitor U0126 and PI3K inhibitor LY294002 induced apoptosis as early as 6 h after addition to cultures. In contrast, addition of the JNK pathway inhibitor SP600125 had little effect on tissue growth. ( d ) Working model of signalling pathways regulated by WT1 in early MM. WT1 induces FGF signalling by directly regulating Fgf16 and Fgf20 gene expression. Binding of FGF to its receptors activates intracellular signalling pathways that induce proliferation and directly suppress pSMAD signalling. In the absence of WT1, loss of FGF signalling and the induction of the BMP/pSMAD signalling pathway leads to widespread apoptosis within the metanephric blastema. Scale bar, 100 μm. Full size image To further delineate the mode of action of FGF induced pSMAD suppression in kidney explants, we used drugs targeting intracellular signalling pathways. As already described above, inhibition of the JNK pathway (SP600125) had little effect on organ growth at least for 24 h ( Fig. 8b,c ). However, when using drugs targeting the Pi3K (LY294002) and MAPK (U0126) pathway, organ cultures stopped growing and underwent apoptosis. Immunostaining confirmed broad upregulation of pSMAD1/5/8, as early as 6 h after treatment. We conclude that activation of FGF signalling is required and sufficient to suppress pSMAD signalling-induced apoptosis in renal explants. ChIP-Seq analysis performed in the present study revealed 36,512 WT1-associated regions, which we limited to 5,547 high-confidence binding regions by setting an IDR cutoff of ≤0.1. The high reproducibility of the peaks in two independent biological experiments suggests that the majority of these sites are indeed occupied by WT1. One reason for the high number of targets might be the use of entire kidneys rather than an isolated cell population as starting material for the ChIP experiments. Indeed the range of WT1-associated genes is diverse and includes genes expressed in renal progenitors, pretubular aggregates and differentiated podocytes, which is in agreement with the multiple functions of WT1 in kidney development. Our ChIP-Seq data therefore provides a rich resource for in-depth investigations on the function of WT1 and the identification of gene regulatory networks governing kidney development. Motif discovery performed on our ChIP-Seq data revealed a WT1 motif that shows high similarity with previously published motifs identified by ChIP-on-Chip experiments [15] . The most striking difference of the new motif is the dominance of an A at position 9. Since, this binding site is highly similar to a sequence identified as a target for the WT1(+KTS) isoform using a whole-genome PCR approach [36] and has since then been confirmed in several promoter-driven studies [37] , [38] , [39] , we are confident that the refined positioned weight matrix represents the bona fide in vivo binding site of WT1. Interestingly, while we observed a significant enrichment close to promoters, the majority of binding sites including the strongest peak mapped rather distant from the TSSs. Thus a major function of WT1 may be to bind to long-distance enhancers or by modifying chromatin structure, as has been recently suggested by Essafi et al . [12] In early kidney development renal progenitors receive vital cues that decide between cell survival and apoptosis. In the present study, we have used WT1 as an entry point to identify events that are at the root of this decision. By combining ChIP-Seq and gene expression profiling of microdissected early metanephric rudiments, we identified a set of renal stem/progenitor cell-specific genes that depend on WT1 expression. A major role for WT1 within this compartment appears to be the regulation of key signalling pathways. Apart from FGF and BMP signalling (discussed below), loss of WT1 appears to influence Wnt/β-catenin signalling, a key pathway in kidney organogenesis [40] . Indeed, we observed a marked reduction of Wnt8b (7.4 × ; P =5.0e−7; Student’s t -test) and Rspo1 (6.3 × ; P =9.5e−9; Student’s t -test) expression. According to Gudmap and Eurexpress databases, Wnt8b expression is relatively low in developing kidneys, and since Wnt8b mutants are phenotypically normal [41] , we did not further investigate its potential role in kidney development. Rspondins encode important regulators of canonical β-catenin signalling by binding to leucine-rich repeat-containing G protein-coupled receptors [42] . Rspo1 knockout mice, however, do not show a renal phenotype [43] , which might be due to persistent expression of other members of the Rspondin gene family, such as Rspo3 . A comprehensive evaluation of the role of Rspondins in renal progenitor cell survival and proliferation will therefore require the generation of conditional Rspo1/3 double-knockout mice. With a 28-fold enrichment score (according to GOrilla analysis), FGF signalling was the most markedly affected annotation cluster in Wt1 mutant mesenchyme. FGFs have been shown previously to play an important role in MM renewal [5] and deletion of Fgfr1 and Fgfr2 within this tissue leads to a phenotype that precisely phenocopies the renal defects seen in Wt1 mutant animals [6] . Accordingly, simultaneous removal of the MM-specific Fgf20 and the Fgf9 leads to renal agenesis in mice [7] . The striking similarities of these severe renal phenotypes suggest that Wt1 gene function and FGF signalling are mechanistically linked during early kidney organogenesis. Here, we demonstrate that WT1 acts at multiple levels within the FGF signalling pathway, and in addition it modulates BMP signalling to ensure survival and maintenance of renal progenitor cells. The following key pieces of evidence support these conclusions. First, Fgf16 and Fgf20 are direct targets of transcriptional regulation by WT1 (ref. 15 and this study) and loss of Wt1 reduces messenger RNA expression of these genes, thus establishing a functional link of these genes. Accordingly, loss of Wt1 also leads to marked reduction of FGF target genes in MM such as Etv5 . Second, WT1 is not only required to induce the FGF pathway within the MM, but at the same time to reduce antagonistic BMP/SMAD signalling. This is evidenced by a massive increase of pSMAD1/5/8 staining in the Wt1 mutant MM and may be partly dependent on Bmper , another target of WT1. Our microarray data further suggest that WT1 action may influence FGF signalling in an indirect manner. FGF signalling requires heparan-sulphate chains at the cell surface of target cells [44] , and kidney organogenesis is critically dependent on heparan-sulphate 2-O-sulphotransferase 1 ( Hs2st1) gene function [45] . Here we identified Hs3st6 , a relative of Hs2st1 , to be subject to WT1 regulation (fourfold; P =8.9e−08; Student’s t -test). Lack of Wt1 within the early MM not only caused loss of FGF gene expression, but also induced ectopic pSMAD signalling, which is a known downstream effector of BMP action. BMP7 has been described as a pro-survival factor for renal progenitor cells [46] , and at later stages it appears to play an important role in priming renal progenitors for subsequent MET [35] . The notion that BMP signalling acts pro-apoptotic may therefore seem at a first glance surprising. However, immunostaining and reporter assays indicate an absence of pSMAD signalling from early renal progenitors [47] , [48] . In vitro experiments suggest that BMP7 promotes progenitor proliferation via a JNK-dependent mechanism [34] . In contrast, increased levels of pSMAD have been reported in apoptotic (E11) MM of mice lacking the BMP modulator Grem1 (ref. 49 ). Rescue of renal agenesis in these mutants has been achieved by genetically reducing BMP levels [48] , [50] thus linking apoptosis with increased BMP signalling. A pro-apoptotic action of pSMAD signalling at later stages of kidney development has also been reported in mice carrying mutations in the phosphatase Dullard , a negative regulator of the pSMAD pathway [51] . Analogously, we argue here that the strong increase of pSMAD in Wt1 −/− MM is a major factor involved in apoptosis of Wt1 mutant mesenchyme. The fact that inhibition of canonical BMP signalling with either recombinant Gremlin or the pharmacological inhibitor dorsomorphin partially rescued the Wt1 Vivo-Morpholino knockdown phenotype strongly supports our model. Surprisingly, our experiments with recombinant BMP4 and BMP7 provoked distinct responses within renal explants: whereas BMP7 treatment had a mild growth-promoting effect, BMP4 caused caspase3 induction and massive cell death, a phenotype that has been observed previously [33] and that is consistent with the pro-apoptotic action of pSMAD signalling in renal progenitor cells. At present we do not know how these differential BMP activities are accomplished, but we hypothesize that the two BMP proteins induce distinct signalling cascades in this setting. Intriguingly, simultaneous inhibition of the JNK pathway effectively converted BMP7 into a pro-apoptotic factor, similar to BMP4. Given these results it may seem surprising, that Bmp4 does not induce renal agenesis, but rather rescues the late (E13.5) renal defects in Bmp7:Bmp4 knock-in mice [52] . We hypothesize that the presence of Fgfs (see below for details), Grem1 and potentially Bmper might be sufficient to direct BMP4 action towards non-canonical, growth-promoting pathways (for example, JNK). Disruption of Grem1 or Wt1 gene functions in vivo or addition of recombinant BMP4 to organ cultures overrides these antagonistic effects, thus leading to activation of pSMAD signalling and MM apoptosis. At later stages during nephrogenesis the cellular response of mesenchymal cells to pSMAD signalling seems to change and BMP7-induced pSMAD is necessary for priming progenitor cells for subsequent MET [35] . Interestingly early CM cells (E11.5) can be induced to undergo MET without BMP7 priming, thus further underlining the distinct properties of renal progenitors at different stages of development. Taken together these data highlight the complexity of BMP signalling, which clearly depends on the cellular context, developmental timing and the presence of pathway modulators, such as BMPER. Future experiments will need to address how these parameters influence the intracellular cascades induced within renal progenitors at different stages of kidney organogenesis. Our data clearly show that FGF and pSMAD signalling induce opposite responses in early MM. The fact that addition of FGF20 suppresses the pro-apoptotic action of BMP4 in kidney organ cultures and rescues apoptosis in Wt1 mutant MM demonstrates that these two signalling pathways act in an antagonistic manner. BMP and FGF signalling have already been shown in other organ systems to act as opposing factors [53] , [54] . Part of this action may involve direct phosphorylation of the SMAD linker region via MAPK pathway, which induces SMAD degradation [55] . Moreover, the marked upregulation of pSMAD1/5/8 after inhibiting FGF signalling with pathway-specific inhibitors, suggests that FGF-mediated suppression of pSMAD is an active process required for normal development. Attenuation of MAPK/PI3K signalling by loss of FGF in Wt1 mutants is therefore likely to increase signalling by stabilizing pSMAD. In addition, the increase of pSMAD signalling in mutant mesenchyme might be partly brought about by the reduced expression of the BMP modulator Bmper , a direct downstream target of WT1, as demonstrated in the present study. BMPER can act both as agonist and antagonist of BMP signalling, and genetic analysis in mice suggests that BMPER enhances the pro-survival function of BMPs in renal progenitors after E13.5 (refs 56 , 57 ). Our in vitro analysis is in line with the notion that BMPER has primarily a suppressive role and prevents BMP4-induced-apoptosis in early kidney development. In summary, our data provide mechanistic insights into the molecular cause of renal agenesis by revealing the existence of two opposing forces, FGF and BMP/pSMAD signalling, acting within the early kidney anlagen ( Fig. 8d ). Bmp4 is expressed in the mesenchyme surrounding the early metanephric blastema [58] and is involved in suppressing ureter outgrowth [48] . Inhibition of the BMP/SMAD pathway and activation of FGF signalling is required to allow survival and proliferation of the specified nephron progenitor cells. WT1 holds a key role in supporting MM survival and proliferation through an FGF-mediated repression of BMP/pSMAD signalling. Mutant mouse strain All animal work was conducted according to national and international guidelines and has been approved by the local ethics committee (CIEPAL NCE/2011-19). Wt1 mutant mice (gift of J. Kreidberg, Harvard, USA) [10] were maintained on a mixed (C57Bl6 crossed with B6DBA/F1) genetic background and genotyped as described previously [59] ( Supplementary Table 1 ). In situ hybridization WISHs were carried out according to ref. 60 . For in situ hybridization on sections, tissues were embedded in paraffin, cut at 10 μm and transferred onto coated glass slides. No signal above background was observed within tissues hybridized with the sense probes. Mouse Gdnf , Ret and Etv5 mouse probes were gifts from F. Costantini (New York). Rspo1 anti-sense probe was synthesized according to ref. 43 . Other ISH probes were amplified from mouse E12.5 wild-type kidney complementary DNA using 5′-AAGACCAAAAAGAACTTCAA-3′ and 5′-GTGATGGTTGACAAAGG-3′ primers for Phf19 , and 5′-TACCCCTTCCCGCCAAGAGA-3′ and 5′-CAGGGAAAAGGTAACGGCGCCT-3′ primers for Hs3st6 . Reverse transcription PCR and qPCR The two renal tissues of E10.25 embryos were surgically microdissected (see Fig. 2a ), pooled and instantly snap frozen at −80 °C. Total RNAs were extracted using Absolutely RNA RT-PCR miniprep kits (Stratagene) and reverse transcription PCR was performed using the M-MLV reverse transcriptase described protocol (Invitrogen). Complementary DNAs were quantified on the ND-1000 Nanodrop and a minimum of 20 ng was used per sample per qPCR. Specific probes and primers for qPCRs were designed on the Roche assay design center website ( www.universalprobelibrary.com ; Supplementary Table 2 ), and quantitative reactions were carried out using the Light Cycler FastStart DNA Master PLUS Hybridization Probes Kit (Roche) for the Gapdh internal standard gene and the Light Cycler TaqMan Master Kit (Roche) for the tested genes. SigmaPlot and GraphPad programs were used for the unpaired t -test statistical analysis with a P <0.01. Immunofluorescence analysis Whole-mount staining: renal tissues were fixed in cold methanol for 20′ and blocked for 2 h in 2% bovine serum albumin (BSA). For primary antibodies and dilutions please see Supplementary Table 3 . Antibodies were diluted in phosphate-buffered saline (PBS)-0.1% Triton and 0.1% BSA. Secondary antibodies including Alexa Fluor 488 anti rabbit, Alexa Fluor 594 anti rabbit, Alexa Fluor 647 anti mouse (all purchased from Life Technology) were used at a dilution of 1:200. Extravidin FITC and streptavidin Cy3 (Sigma) were diluted to 1:300. Immunofluorescence staining on cryosections was performed as follows: embryos were fixed in Antigen fix (Microm Microtech) for 2 h, incubated in 30% sucrose overnight then embedded in Tissue-Tek O.C.T. Compound (Sakura) and cut at 8 μm. Cryosections were blocked in 5% normal goat serum, 1% BSA and 0.1% Triton. TUNEL staining For cell death detection in whole-kidney explants, tissues were fixed for 20 min in methanol. TUNEL assays were performed according to the manufacturer’s instructions (In Situ Cell Death Detection Kit, TMR red, Roche). For cell death detection on sections, tissues were fixed in 4% paraformaldehyde, paraffin embedded and sectioned at 10 μm. The sections were transferred onto gelatine-coated slides and apoptotic cell death was detected according to the manufacturer’s instructions. Genetic deletion of Wt1 in organ cultures The Wt1 flox allele was crossed with Wt1 CreERT2 mice and kidneys isolated from E11.5 embryos. Genetic deletion was induced by addition of 4-OH-tamoxifen (2 μM) to the culture medium. For rescue experiments, the medium was further supplemented with FGF growth factors (see Supplementary Table 4 for concentrations). Kidney rudiments were analysed after 48 h in culture. ChIP-Seq and bioinformatic analysis Kidneys were dissected from E18.5 mouse embryos and diced in ice-cold Hanks buffered saline solution. ChIP was performed essentially as described in ref. 61 with modifications to cell lysis and sonication steps as follows. After fixation, tissue was disrupted and nuclei released by homogenization in a 15-ml Potter S homogenizer with Teflon plunger (B. Braun) attached to a drill in 20 mM HEPES pH 7.4, 1 mM EDTA, 150 mM NaCl, 1% SDS, 0.125 M glycine, 0.2 mg ml −1 PMSF. Nuclei were collected by centrifugation (805 g for 5 min) and re-suspended for sonication in 20 mM HEPES pH 7.4, 1 mM EDTA, 150 mM NaCl, 0.4% SDS, 0.2 mg ml −1 PMSF. Chromatin was fragmented to an average length of 600 bp. 3 μg of WT1 antibody (Santa Cruz C-19, sc-192), or IgG were used for immunoprecipitation. For ChIP-Seq library preparation, recovered DNA was digested with either AluI/MseI or HaeIII/MseI . Ends were filled and fragments A-tailed by treatment with GoTaq (Promega). Forked adapters (Illumina genomic DNA sample prep kit) were ligated to fragments and the resulting product was subject to 18 rounds of amplification using Illumina PCR primers and Pfx DNA polymerase (Invitrogen). Library concentration and fragment size were determined on an Agilent Bioanalyzer. Typically, from 5 ng of input this method produced 900 ng of library with an average size of 400 bp. Libraries were sequenced on Illumina Genome Analyzer (GAII, MDC, Berlin). Two independent experiments were carried out and mapped to the mouse genome (mm10). Analysis was carried out using MACS1.4 keeping duplicates [62] or the GENOMATIX software suite using the two independent experiments as biological replicates (details on request). Peak regions from both replicates were integrated using IDR analysis [16] and high confidence binding regions with IDR cutoff below 0.01 were subjected to de novo motif discovery using MEME-ChIP v4.9.1_1 (ref. 17) [17] restricting the maximum motif width to 12 base pairs. Motif comparison was performed against a database of pooled TF motifs [63] , [64] , [65] and the previously discovered motif for WT1 (ref. 15) [15] . Functional annotation of high confidence binding regions was performed using Genomic Regions Enrichment of Annotations Tool (GREAT) [18] . Custom scripts (see Supplementary Software 1 ) were used to integrate ChIP-Seq and differential gene expression analysis. For visual inspection of WT1 binding to specific genomic regions ( Figs 3a and 5a ), normalized read densities (wig files) were uploaded to the UCSC genome browser and the identical viewing range for both WT1 and control samples set to the maximum peak within the window. Microarray study and data processing Total RNA was extracted from microsurgically dissected metanephric kidneys of knockout and heterozygous E10.25 (tail somite 8–13) embryos using the RNeasy MicroKit (Qiagen) followed by column DNase digestion to remove any contaminating genomic DNA. For microarray analysis 4 independent pools for each genotype were prepared by combining RNA from 16 kidneys (8 embryos) for each pool (sample). Labelling of cRNA, microarray hybridization and image processing was carried out according to manufacturers’ instructions (Applied Biosystems 1,700 chemiluminescent microarray analyzer). To identify differentially expressed genes in the Wt1 heterozygous and knockout mice, the raw gene expression data values were pre-processed for multiarray analysis using Gene Spring GX software (Version 7.3.1; Agilent technologies). This was followed by per-chip median polishing and per-gene normalization to specific samples. Statistical analysis was performed using Welch parametric t -test on genes given as present calls (P calls) and using a P -value equal or less than 0.05 as a measure of significance for differential expression ( Supplementary Data 4 ). For gene enrichment analysis, the ranked gene list was uploaded to GOrilla and analysed using ‘Function’ as an ontology setting. For the gene lists of down- and upregulated genes presented in Supplementary Data 4 (worksheet 2 and 3) a raw data value of 1,000 was set as a cutoff threshold to reduce genes with extremely low levels of expression. Organ cultures Kidney rudiments were microsurgically isolated from E11.5 wild-type embryos (SWISS Webster, purchased from Charles River) in 1 × PBS and kept on ice until they were transferred to culture dishes. They were then transferred to polycarbonate membranes (0.5-μm pore size, Whatman) supported by a metal grid in 24-well dishes containing 200 μl of MEM Eagle (Gibco) supplemented with 10% newborn calf serum (Gibco), 2 mM glutamine (Gibco) and 0.5% penicillin-streptomycin (Gibco). Kidneys were incubated for 42 to 72 h without replacing the medium. For gene knockdown assays, Vivo-Morpholinos (Gene Tools, LLC) at a concentration of 5 μM ( Wnt4 ) or 7.5 μM ( Wt1 ) were directly added to the medium. For rescue experiments, media were further supplemented with recombinant proteins or pathway inhibitors ( Supplementary Table 4 ). For sequences of Vivo-Morpholinos please see Supplementary Table 5 . Ureteric bud tips were counted manually after staining with calbindin, cytokeratin or lectin. Quantification of apoptotic cells and nascent epithelia was performed by automatic counting (Image J) of caspase3- and JAG1-positive cells, respectively. MM cultures E11.5 MM was separated from UB by incubation of kidney rudiments in 3% pancreatin/trypsin (Gibco-BRL) in PBS. MM cells were cultured (one kidney per well) on a 24-well plate coated with ECM gel (Sigma) in 5% fetal calf serum medium or free serum media supplemented by FGF2 (50 ng ml −1 ) and transforming growth factor alpha (20 ng ml −1 ). After 72 h of culture the cells were washed and starved for 5 or 10 h before adding FGF20 (5 ng ml −1 ) to the medium. How to cite this article: Jian Motamedi, F. et al . WT1 controls antagonistic FGF and BMP-pSMAD pathways in early renal progenitors. Nat. Commun. 5:4444 doi: 10.1038/ncomms5444 (2014). Accession codes : Microarray and sequencing data have been deposited in GEO under accession number GSE58073 and GSE58179 , respectively.